Greatwall kinase and cyclin B-Cdk1 are both critical constituents of M-phase-promoting factor Maturation/M-phase-promoting factor is the universal inducer of M-phase in eukaryotic cells. It is currently accepted that M-phase-promoting factor is identical to the kinase cyclin B–Cdk1. Here we show that cyclin B–Cdk1 and M-phase-promoting factor are not in fact synonymous. Instead, M-phase-promoting factor contains at least two essential components: cyclin B–Cdk1 and another kinase, Greatwall kinase. In the absence of Greatwall kinase, the M-phase-promoting factor is undetectable in oocyte cytoplasm even though cyclin B–Cdk1 is fully active, whereas M-phase-promoting factor activity is restored when Greatwall kinase is added back. Although the excess amount of cyclin B–Cdk1 alone, but not Greatwall kinase alone, can induce nuclear envelope breakdown, spindle assembly is abortive. Addition of Greatwall kinase greatly reduces the amount of cyclin B–Cdk1 required for nuclear envelope breakdown, resulting in formation of the spindle with aligned chromosomes. M-phase-promoting factor is thus a system consisting of one kinase (cyclin B–Cdk1) that directs mitotic entry and a second kinase (Greatwall kinase) that suppresses the protein phosphatase 2A-B55 which opposes cyclin B–Cdk1. MPF (maturation/M-phase-promoting factor) is now used as the term for the universal inducer of entry into M-phase throughout eukaryotic cells [1] , [2] . MPF was originally identified by a functional assay in vertebrate and invertebrate oocyte systems. Immature oocytes arrest their cell cycle at the G2/M-phase border in the first meiosis [3] . This arrest is released by a maturation-inducing hormonal stimulus at the oocyte surface. MPF was first described as 'maturation-promoting factor', that is, a cytoplasmic activity of hormone-treated maturing oocytes that upon transfer causes recipient immature oocytes to undergo the meiotic G2/M-phase transition without hormonal stimulation [4] , [5] . Thereafter, a similar transferable activity that can induce the meiotic G2/M-phase transition in recipient oocytes was demonstrated in M-phase extracts of mitotic somatic cells from yeast to mammals [6] , [7] , [8] , [9] . MPF was thus renamed 'M-phase-promoting factor' to imply that it is an M-phase inducer common to all eukaryotic cells. By the end of the 1980s, three separate lines of research on MPF, Cdc2 and cyclin converged to ascribe the M-phase-inducing activity contained in MPF to a particular Ser/Thr kinase, the cyclin B–Cdc2/Cdk1 complex [1] , [2] . Indeed, purified cyclin B–Cdk1 can induce the meiotic G2/M-phase transition upon injection into immature oocytes [10] , [11] , [12] , [13] . If MPF is indeed identical to cyclin B–Cdk1, the levels of purified cyclin B–Cdk1 required for induction of the meiotic G2/M-phase transition in injected immature oocytes should be similar to the amount of cyclin B–Cdk1 found in the original MPF from donor cytoplasm. Surprisingly, however, no such quantitative comparison has yet been performed. After the discovery of the cyclin B–Cdk1 complex, various other mitotic kinases have been identified [14] , and emerging studies indicate that entry into mitosis is controlled by highly coordinated activities between multiple protein kinases and opposing protein phosphatases [15] . The major protein phosphatase that has anti-mitotic activity against cyclin B–Cdk1-directed phosphorylations is the heterotrimeric protein phosphatase 2A that contains a regulatory subunit of the B55 family (PP2A-B55) [16] , [17] . PP2A-B55 is turned off when cyclin B–Cdk1 is turned on, and the key link between these is mediated by the Greatwall kinase (Gwl) [16] , [18] , which was originally identified as Scant (Scott of the Antarctic) in the fruit fly Drosophila [19] . It was later renamed as Gwl and described as a nuclear protein required for proper chromosome condensation and M-phase progression in Drosophila [20] . Gwl is activated downstream of cyclin B–Cdk1 (ref. 21 ), and accomplishes inhibition of PP2A-B55 indirectly through phosphorylation of the small protein α-endosulfine (Ensa) [22] and/or its close relative cyclic adenosine monophosphate-regulated phosphoprotein 19 (Arpp19) [23] . Even though cyclin B–Cdk1 clearly bears the major catalytic activity of MPF, an intriguing possibility is that MPF also involves suppression of the anti-cyclin B–Cdk1 phosphatase (that is, PP2A-B55) through action of Gwl. Here we show that Gwl is in fact a critical constituent of the classically described maturation-promoting factor, in that Gwl can reduce the requirement for cyclin B–Cdk1 to physiological levels to ensure assembly of the spindle. Cyclin B–Cdk1 is not identical to MPF To re-examine the relationship of MPF with cyclin B–Cdk1, we took advantage of the oocytes of frog [4] and starfish [5] in which MPF was first identified. In these oocytes, cyclin B–Cdk1 is activated in response to a maturation-inducing hormone: progesterone [24] for frog and 1-methyladenine (1-MeAde) [25] for starfish. Hormone treatment results in nuclear envelope breakdown (NEBD; also called germinal vesicle breakdown, or GVBD), a clear hallmark of the meiotic G2/M-phase transition. During this transition, the activity of cyclin B–Cdk1 is regulated positively by Cdc25 and negatively by Myt1; cyclin A and Wee1 are both absent at this time and only begin to be newly synthesized at later stages of meiosis [3] . As a source of MPF, so-called cytostatic factor (CSF) extracts were prepared from mature frog oocytes arrested at metaphase of meiosis II (ref. 26 ), or alternatively the cytoplasm was aspirated into a micropipette after GVBD from mature starfish oocytes at metaphase of meiosis I (meta-I) [5] . Cyclin B–Cdk1 was purified from meta-I starfish oocytes [27] . Various amounts of these samples were injected into immature oocytes of frog ( Fig. 1a ) or starfish ( Fig. 1b ) to perform dose-response assays for induction of the meiotic G2/M-phase transition (that is, M-phase-inducing activity). The quantitative comparison indicates that the level of Cdk1 activity required for M-phase entry is roughly one order of magnitude higher when using purified cyclin B–Cdk1 than when using either frog ( Fig. 1a ) or starfish ( Fig. 1b ) oocyte cytoplasmic MPF. Thus, purified cyclin B–Cdk1 can induce the meiotic G2/M-phase transition only when added in great excess with respect to endogenous levels in oocytes. 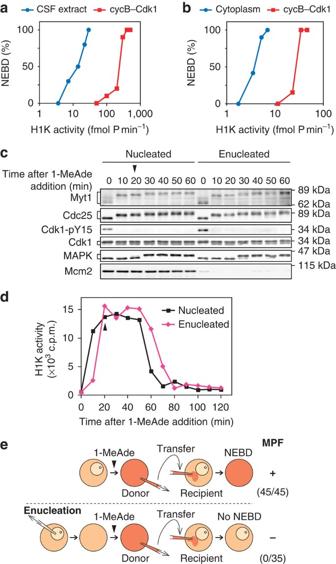Figure 1: Cyclin B–Cdk1 (cycB–Cdk1) is not identical to MPF in either frog or starfish oocytes. (a,b) Purified cycB–Cdk1 requires higher H1K activity for the meiotic G2/M-phase transition than does cytoplasmic MPF. H1K activity required for NEBD induction after injection into recipients was compared inXenopusoocytes between CSF extracts (MPF) and purified cycB–Cdk1 (a), and in starfish oocytes between maturing oocyte cytoplasm (MPF) and purified cycB–Cdk1 (b). H1K activity in the abscissa was calculated from an injection volume and an activity that catalyses the transfer of phosphate from ATP to histone H1 per minute per volume (Methods). (c,d) Enucleated, as well as nucleated, starfish oocytes respond to 1-MeAde by undergoing changes in phosphorylation of Cdc25, Myt1, Cdk1, and MAPK (c), and an increase in cycB–Cdk1 activity, as measured by H1K (d). Mcm2 is a marker for nucleated oocytes. The lower band of Cdk1 corresponds to its Tyr15-dephosphorylated, active form. The upper band of MAPK corresponds to its active form. NEBD (arrow head) occurred at 18–20 min in nucleated oocytes. (e) Cytoplasm from enucleated starfish oocytes exhibits no MPF activity. Cytoplasm (250 pl) of nucleated or enucleated oocytes during metaphase of meiosis I (nucleated) or the equivalent period after 1-MeAde addition (enucleated) was injected into recipient immature oocytes, and NEBD was inspected (numbers with NEBD/total recipients). Figure 1: Cyclin B–Cdk1 (cycB–Cdk1) is not identical to MPF in either frog or starfish oocytes. ( a , b ) Purified cycB–Cdk1 requires higher H1K activity for the meiotic G2/M-phase transition than does cytoplasmic MPF. H1K activity required for NEBD induction after injection into recipients was compared in Xenopus oocytes between CSF extracts (MPF) and purified cycB–Cdk1 ( a ), and in starfish oocytes between maturing oocyte cytoplasm (MPF) and purified cycB–Cdk1 ( b ). H1K activity in the abscissa was calculated from an injection volume and an activity that catalyses the transfer of phosphate from ATP to histone H1 per minute per volume (Methods). ( c , d ) Enucleated, as well as nucleated, starfish oocytes respond to 1-MeAde by undergoing changes in phosphorylation of Cdc25, Myt1, Cdk1, and MAPK ( c ), and an increase in cycB–Cdk1 activity, as measured by H1K ( d ). Mcm2 is a marker for nucleated oocytes. The lower band of Cdk1 corresponds to its Tyr15-dephosphorylated, active form. The upper band of MAPK corresponds to its active form. NEBD (arrow head) occurred at 18–20 min in nucleated oocytes. ( e ) Cytoplasm from enucleated starfish oocytes exhibits no MPF activity. Cytoplasm (250 pl) of nucleated or enucleated oocytes during metaphase of meiosis I (nucleated) or the equivalent period after 1-MeAde addition (enucleated) was injected into recipient immature oocytes, and NEBD was inspected (numbers with NEBD/total recipients). Full size image We further verified that normal endogenous levels of cyclin B–Cdk1 alone are insufficient to induce the G2/M-phase transition in recipient oocytes. Starfish oocytes are optically transparent, and hence the nucleus (called the germinal vesicle, GV) can be easily removed by suction of nuclear contents into a microinjection pipette [28] . In enucleated as well as nucleated oocytes, 1-MeAde stimulus induced electrophoretic mobility shifts of various M-phase regulators, including Myt1 (ref. 29 ), Cdc25 (ref. 27 ), Cdk1 (refs 27 , 29 ) and mitigen-activated protein kinase (MAPK) [30] ( Fig. 1c ). These changes reflect inactivation of Myt1 and activation of Cdc25, Cdk1 and MAPK. Consistently, an increase and subsequent decrease in cyclin B–Cdk1 activity, which represent resumption and completion of meiosis I, respectively, were observed in oocyte lysates ( Fig. 1d ). Although a slight delay occurred in the timing, no difference was detectable in the elevated levels of cyclin B–Cdk1 activity between enucleated and nucleated oocytes. Nevertheless, in contrast to the case of nucleated oocytes, MPF was undetectable in 1-MeAde-treated enucleated oocytes when their cytoplasm was transferred to immature recipients ( Fig. 1e ; refs 31 , 32 ). Adding back the nuclear contents to the enucleated oocyte cytoplasm restores MPF [31] , [32] . Thus, cyclin B–Cdk1 cannot be identical to MPF (see also refs 33 , 34 ). Unless cyclin B–Cdk1 is greatly overexpressed, it needs another factor to function as MPF. This factor must be specifically located in the nucleus of starfish oocytes before GVBD, but then is dispersed in the cytoplasm when the nuclear envelope breaks down at the G2/M transition. MPF is undetectable in the absence of Gwl To identify this missing factor that is required for MPF in addition to cyclin B–Cdk1, we have considered the idea that it is a nuclear component in starfish oocytes. Although the well-known mitotic kinases Plk1 (ref. 35 ), Aurora [36] and MAPK [30] were obvious candidates, these three kinases are not always nuclear. Furthermore, MPF remained detectable when the activities of these kinases were inhibited by drugs in donor oocytes ( Supplementary Table S1 ). Another alternative was suggested by previous studies showing that okadaic acid, an inhibitor of PP2A and PP1, mimics the nuclear component required for MPF [37] , [38] . This finding prompted us to investigate Gwl, because Gwl has been reported both to be localized to the nucleus and to have a role in PP2A inhibition [16] , [18] , [20] . We first isolated a cDNA of the starfish homologue of Gwl ( Supplementary Fig. S1 and Supplementary Methods ) and raised antibodies separately against its amino- and carboxy-terminal kinase domains ( Supplementary Fig. S2a ). Gwl was present in immature starfish oocytes; its protein level remained constant during meiotic and cleavage cycles, whereas it was hyperphosphorylated after meiotic reinitiation ( Fig. 2a ). Gwl was activated (as measured by kinase activity against the model substrate myelin basic protein) following activation of cyclin B–Cdk1 at the meiotic G2/M-phase transition, and thereafter, Gwl activity fluctuated along with the cell cycle. Comparison of quantified kinase activities between H1 kinase (H1K) and Gwl raises the possibility that suppression of PP2A-B55 by Gwl might be more important for phosphorylation of Cdk1 substrates in meiosis II than in mitosis. Both hyperphosphorylation and activation of Gwl at the meiotic G2/M-phase transition depended on cyclin B–Cdk1 activity ( Fig. 2b ). Comparison between nucleated and enucleated immature starfish oocytes indicated that Gwl is exclusively present in the nucleus ( Fig. 2c ). 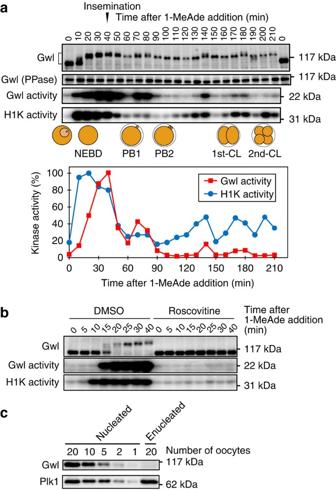Figure 2: Gwl is present exclusively in the nucleus and is activated downstream of cyclin B–Cdk1 at meiotic resumption in starfish oocytes. (a) Gwl kinase activity cycles in parallel with Cdk1 (H1K) activity during meiotic and cleavage cycles. Immature oocytes were treated with 1-MeAde, followed by insemination 40 min later. After immunoprecipitation, Gwl kinase activity was assayed by phosphorylation of myelin basic protein (MBP). To compare amounts of Gwl proteins, oocyte extracts were treated with λ-protein phosphatase (PPase). Quantified activities of H1K and Gwl (normalized to its protein levels) are shown at the bottom. (b) Gwl activation after 1-MeAde treatment does not occur in the presence of the Cdk1 inhibitor, roscovitine. Dimethylsulphoxide (DMSO) indicates the control without roscovitine. (c) Amounts of Gwl protein were compared with immunoblots between the indicated numbers of nucleated or enucleated immature oocytes. Plk1 is a cytoplasmic marker. Figure 2: Gwl is present exclusively in the nucleus and is activated downstream of cyclin B–Cdk1 at meiotic resumption in starfish oocytes. ( a ) Gwl kinase activity cycles in parallel with Cdk1 (H1K) activity during meiotic and cleavage cycles. Immature oocytes were treated with 1-MeAde, followed by insemination 40 min later. After immunoprecipitation, Gwl kinase activity was assayed by phosphorylation of myelin basic protein (MBP). To compare amounts of Gwl proteins, oocyte extracts were treated with λ-protein phosphatase (PPase). Quantified activities of H1K and Gwl (normalized to its protein levels) are shown at the bottom. ( b ) Gwl activation after 1-MeAde treatment does not occur in the presence of the Cdk1 inhibitor, roscovitine. Dimethylsulphoxide (DMSO) indicates the control without roscovitine. ( c ) Amounts of Gwl protein were compared with immunoblots between the indicated numbers of nucleated or enucleated immature oocytes. Plk1 is a cytoplasmic marker. Full size image To determine the role of Gwl, we inhibited Gwl activity using an antibody against Gwl's carboxy terminus. As we could not inject a sufficient amount of antibody directly into the nucleus to suppress Gwl activity ( Supplementary Fig. S2b,c ), we developed a system to deliver IgG to the nucleus after its injection into the cytoplasm. We thus constructed ZZ-IBB, which is composed of two synthetic 'Z' domains derived from the IgG-binding domain of protein A [39] , as well as the nuclear localization signal IBB (importin β-binding domain of importin α) [40] ( Fig. 3a ). In a test of this system, IgG together with ZZ-IBB, but not IgG alone, efficiently entered and accumulated in the nucleus after cytoplasmic injection ( Fig. 3b ), indicating that ZZ-IBB can be used to introduce IgG into the nucleus. Indeed, when the anti-carboxy-terminal Gwl antibody was injected together with ZZ-IBB into the cytoplasm of immature oocytes, Gwl activity remained suppressed after 1-MeAde treatment ( Fig. 3c and Supplementary Fig. S2d ). In these oocytes, NEBD nonetheless occurred with only a slight delay after 1-MeAde addition ( Fig. 3d ). Consistently, electrophoretic mobility shifts of various M-phase regulators, including Myt1, Cdc25 and MAPK, and activation of cyclin B–Cdk1 occurred almost normally, although a slight delay in these parameters was observed ( Fig. 3e ). Thus, Gwl is apparently dispensable for the meiotic G2/M-phase transition transition after 1-MeAde-induction (Discussion). 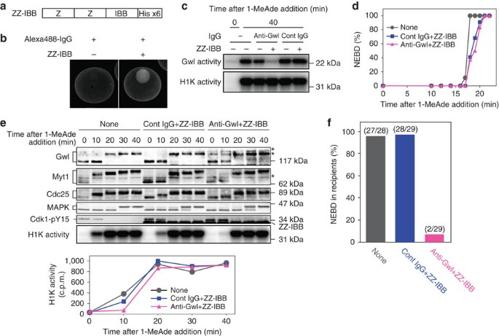Figure 3: Gwl is necessary for MPF in starfish oocytes. (a,b) ZZ-IBB causes nuclear accumulation of IgG. Schematic diagram of the ZZ-IBB construct (a). Immature oocytes were injected with fluorescently labelled donkey IgG (Alexa488-IgG) in the absence or presence of ZZ-IBB, and then examined by confocal microscopy (b). (c) Anti-Gwl-C antibody (anti-Gwl) along with ZZ-IBB inhibits activity of Gwl, but not cyclin B–Cdk1. Immature oocytes, which had been injected with either anti-Gwl or control IgG in the absence or presence of ZZ-IBB, were treated with 1-MeAde, followed by examination of Gwl and Cdk1 (H1K) activities at 40 min. (d,e) Gwl is not essential for meiotic resumption. Gwl-inhibited oocytes, which had been injected with anti-Gwl along with ZZ-IBB, were treated with 1-MeAde. Thereafter, the time courses of NEBD (d) and Cdk1 activation (e), and changes in the phosphorylations of Gwl, Cdc25, Myt1, Cdk1 and MAPK (e) were monitored. Asterisks indicate non-specific bands. (f) MPF is undetectable from Gwl-inhibited oocytes. For MPF assay, cytoplasm from Gwl-inhibited and 1-MeAde-treated oocytes (anti-Gwl+ZZ-IBB), from control IgG-injected and 1-MeAde-treated oocytes (Cont IgG+ZZ-IBB), or from oocytes treated with 1-MeAde alone (None) was transferred into immature oocytes in which NEBD was inspected (numbers with NEBD/total recipients). Figure 3: Gwl is necessary for MPF in starfish oocytes. ( a , b ) ZZ-IBB causes nuclear accumulation of IgG. Schematic diagram of the ZZ-IBB construct ( a ). Immature oocytes were injected with fluorescently labelled donkey IgG (Alexa488-IgG) in the absence or presence of ZZ-IBB, and then examined by confocal microscopy ( b ). ( c ) Anti-Gwl-C antibody (anti-Gwl) along with ZZ-IBB inhibits activity of Gwl, but not cyclin B–Cdk1. Immature oocytes, which had been injected with either anti-Gwl or control IgG in the absence or presence of ZZ-IBB, were treated with 1-MeAde, followed by examination of Gwl and Cdk1 (H1K) activities at 40 min. ( d , e ) Gwl is not essential for meiotic resumption. Gwl-inhibited oocytes, which had been injected with anti-Gwl along with ZZ-IBB, were treated with 1-MeAde. Thereafter, the time courses of NEBD ( d ) and Cdk1 activation ( e ), and changes in the phosphorylations of Gwl, Cdc25, Myt1, Cdk1 and MAPK ( e ) were monitored. Asterisks indicate non-specific bands. ( f ) MPF is undetectable from Gwl-inhibited oocytes. For MPF assay, cytoplasm from Gwl-inhibited and 1-MeAde-treated oocytes (anti-Gwl+ZZ-IBB), from control IgG-injected and 1-MeAde-treated oocytes (Cont IgG+ZZ-IBB), or from oocytes treated with 1-MeAde alone (None) was transferred into immature oocytes in which NEBD was inspected (numbers with NEBD/total recipients). Full size image Surprisingly, however, MPF was undetectable from these Gwl-inhibited oocytes. As assayed by cytoplasmic transfer, cytoplasm from oocytes that were both Gwl-inhibited and 1-MeAde-treated exhibited no M-phase-inducing activity in recipients, in contrast with cytoplasm from control donors ( Fig. 3f ). Gwl is thus required for MPF even in the presence of normal levels of cyclin B–Cdk1 activity. Gwl restores MPF As enucleation and inhibition of nuclear Gwl activity induced very similar effects, we then added back Gwl into enucleated starfish oocytes to examine if this treatment could restore MPF. Recombinant wild-type (rGwl-WT) or kinase-deficient mutant protein (rGwl-G52S) was injected into enucleated oocytes to introduce approximately the same amount of Gwl as in nucleated oocytes ( Fig. 4a and Supplementary Fig. S3 ). After treatment with 1-MeAde, cyclin B–Cdk1 was activated and an electrophoretic mobility shift of the rGwls was seen, suggesting activation of rGwl-WT in enucleated oocytes ( Fig. 4a ). MPF was detectable from enucleated oocytes that had received injection of WT-, but not G52S-, rGwl ( Fig. 4b ). Furthermore, injection of purified active rGwl-WT along with cytoplasm from enucleated, 1-MeAde-treated oocytes exhibited MPF in recipients, whereas active rGwl-WT alone exhibited no MPF function even at sevenfold higher levels of kinase activity ( Fig. 4c ). Thus, Gwl activity is sufficient to restore MPF in enucleated oocytes treated with 1-MeAde, even though Gwl by itself is devoid of MPF activity. Although Gwl alone has been reported to be able to induce the meiotic G2/M-phase transition in frog oocytes without hormone treatment [41] , this effect was observed only when pre-activated Gwl was injected at much higher than endogenous levels. 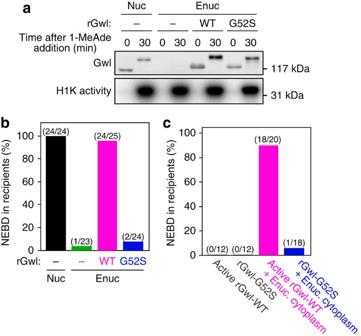Figure 4: Gwl restores MPF in enucleated starfish oocytes. (a,b) Gwl is sufficient for restoration of MPF in enucleated oocytes (Enuc). Enuc were injected with recombinant Gwl protein (rGwl-WT) or its kinase-dead mutant (rGwl-G52S), in the same amounts as the endogenous Gwl in an oocyte (0.06 fmol). These oocytes and control nucleated (Nuc) or Enuc oocytes were treated with 1-MeAde, and then examined for the amount of Gwl protein (upper) and the level of H1K (lower) at the indicated times (a), or for MPF activity by cytoplasmic transfer into immature oocytes (numbers with NEBD/total recipients) (b). (c) Gwl together with the cytoplasm of 1-MeAde-treated enucleated oocytes, but not Gwl alone, exhibits MPF activity. Immature oocytes were injected with 1.2 fmol of active rGwl-WT, whose activity is sevenfold higher than that of the total endogenous Gwl in a meta-I oocyte; but no NEBD occurred (active rGwl-WT). In contrast, immature oocytes were injected with 250 pl of cytoplasm from an enucleated, 1-MeAde-treated oocyte along with 14 amol of active rGwl-WT, whose activity is equivalent to the endogenous Gwl in 250 pl of cytoplasm from a nucleated, meta-I oocyte; and then NEBD occurred (active rGwl-WT+Enuc cytoplasm). As controls, the same amounts of kinase-dead rGwl-G52S, with or without cytoplasm from Enuc and 1-MeAde-treated oocytes, were injected. In parentheses, numbers with NEBD/total recipients. Figure 4: Gwl restores MPF in enucleated starfish oocytes. ( a , b ) Gwl is sufficient for restoration of MPF in enucleated oocytes (Enuc). Enuc were injected with recombinant Gwl protein (rGwl-WT) or its kinase-dead mutant (rGwl-G52S), in the same amounts as the endogenous Gwl in an oocyte (0.06 fmol). These oocytes and control nucleated (Nuc) or Enuc oocytes were treated with 1-MeAde, and then examined for the amount of Gwl protein (upper) and the level of H1K (lower) at the indicated times ( a ), or for MPF activity by cytoplasmic transfer into immature oocytes (numbers with NEBD/total recipients) ( b ). ( c ) Gwl together with the cytoplasm of 1-MeAde-treated enucleated oocytes, but not Gwl alone, exhibits MPF activity. Immature oocytes were injected with 1.2 fmol of active rGwl-WT, whose activity is sevenfold higher than that of the total endogenous Gwl in a meta-I oocyte; but no NEBD occurred (active rGwl-WT). In contrast, immature oocytes were injected with 250 pl of cytoplasm from an enucleated, 1-MeAde-treated oocyte along with 14 amol of active rGwl-WT, whose activity is equivalent to the endogenous Gwl in 250 pl of cytoplasm from a nucleated, meta-I oocyte; and then NEBD occurred (active rGwl-WT+Enuc cytoplasm). As controls, the same amounts of kinase-dead rGwl-G52S, with or without cytoplasm from Enuc and 1-MeAde-treated oocytes, were injected. In parentheses, numbers with NEBD/total recipients. Full size image Gwl reduces MPF's requirement for cyclin B–Cdk1 The above observations identify Gwl as a nuclear component necessary for MPF in starfish oocytes. Nonetheless, it is well known that purified cyclin B–Cdk1 has MPF activity [12] , [13] . A possible clue to reconcile these findings is the observation that considerable overexpression is required for cyclin B–Cdk1 alone to function as MPF ( Fig. 1a,b ). We thus asked whether Gwl can reduce the amount of cyclin B–Cdk1 activity that is required for MPF both in starfish and frog oocytes. To perform quantitative analysis in the starfish oocyte system, the amount of Gwl protein was estimated by western blotting to be 60 amol in a single oocyte (volume, 3.0 nl; Supplementary Fig. S3c ). Accordingly, the 105 pl of cytoplasmic MPF, which was able to induce 50% NEBD in a recipient oocyte, contains 2.1 amol of Gwl protein ( Fig. 5a ). In terms of the kinase activity, 2.1 amol of Gwl was equivalent to 6.1 amol of the active rGwl-WT due to low specific activity of recombinant Gwl ( Supplementary Fig. S3b,c ). Immature oocytes were then injected with various activity levels of purified cyclin B–Cdk1 along with or without 6.1 amol of the active rGwl-WT (that is, a kinase level equivalent to that in MPF) to measure the dose of purified cyclin B–Cdk1 for induction of the meiotic G2/M-phase transition ( Fig. 5b ). Addition of active Gwl greatly reduced the amount of cyclin B–Cdk1 activity required for MPF by about 75% (that is, from 25.1 to 6.12 fmol P min −1 for 50% NEBD induction; Fig. 5b,c ). Thus, Gwl contributes to MPF by reducing the required amount of cyclin B–Cdk1 activity.As for a reason for this reduction, one possibility could be that Gwl could directly enhance the kinase activity of cyclin B–Cdk1. However, this is unlikely, because at injection into recipient oocytes, rGwl and purified cyclin B–Cdk1 were separated in a micropipette (Methods) and hence had no opportunity to mix. In addition, the levels of histone H1K activity in oocytes were not affected by the presence or absence of nucleus (that is, Gwl) after 1-MeAde addition ( Fig. 1d ); and finally, in vitro mixing of purified cyclin B–Cdk1 with active rGwl did not affect the H1K activity of cyclin B–Cdk1 ( Supplementary Fig. S4 ; Discussion). 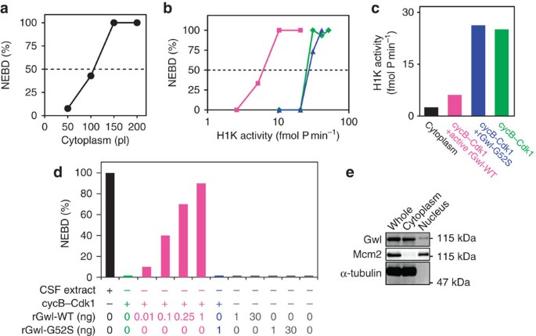Figure 5: Cyclin B–Cdk1 (cycB–Cdk1) plus Gwl is nearly identical to MPF in starfish and frog oocytes. (a) In starfish, various volumes of cytoplasm from maturing oocytes were injected into immature oocytes, and the volume of cytoplasm that induces NEBD in 50% of recipients was estimated to be 105 pl. This volume of cytoplasm was calculated to contain Gwl activity equivalent to 6.1 amol of active rGwl-WT (see Methods in detail) and an H1 kinase (H1K) activity of 2.56 fmol P min−1(Methods; for below (c)). (b) Gwl reduces the dose dependence of cycB–Cdk1 for NEBD induction in starfish oocytes. Various amounts of purified cycB–Cdk1, having kinase activities of 2.5–50 fmol P min−1(each dissolved in a volume of 100 pl; Methods), were injected into immature oocytes along with (magenta squares) or without (green diamonds) active rGwl-WT (6.1 amol in 35 pl solution; see (a) above). Kinase defective rGwl-G52S (blue triangles) was used as a control. (c) Supplementation of purified cycB–Cdk1 with the endogenous level of Gwl reduced the level of cycB–Cdk1 required for NEBD induction in starfish oocytes by ~75% (from 25.1 to 6.12 fmol P min−1). From graphs (a,b), the amounts of H1K activity required for 50% NEBD were estimated. (d) Supplementation with Gwl transforms cycB–Cdk1 to MPF inXenopusoocytes. For MPF assay, immature oocytes were injected with purified cycB–Cdk1 at a level of H1K activity, which is insufficient for NEBD induction (60 fmol P min−1in 0.23 nl), without (green) or with various amounts of active rGwl-WT (magenta, 0.01–1.0 ng in 2.1 nl) or control kinase defective rGwl-G52S (blue, 1.0 ng in 2.1 nl). Neither rGwl-WT nor rGwl-G52S alone (gray, 1.0 or 30 ng in 2.1 nl) induced NEBD. As a positive control, CSF extract (black; H1K activity, 60 fmol P min−1in 18.4 nl) invariably induced NEBD. (e) Gwl is localized mostly in the cytoplasm of immatureXenopusoocytes. Amounts of Gwl were compared by immunoblotting among whole immature oocytes (whole), enucleated immature oocytes (cytoplasm) and isolated GVs (nucleus). Mcm2 and α-tubulin are nuclear and cytoplasmic markers, respectively. Figure 5: Cyclin B–Cdk1 (cycB–Cdk1) plus Gwl is nearly identical to MPF in starfish and frog oocytes. ( a ) In starfish, various volumes of cytoplasm from maturing oocytes were injected into immature oocytes, and the volume of cytoplasm that induces NEBD in 50% of recipients was estimated to be 105 pl. This volume of cytoplasm was calculated to contain Gwl activity equivalent to 6.1 amol of active rGwl-WT (see Methods in detail) and an H1 kinase (H1K) activity of 2.56 fmol P min −1 (Methods; for below ( c )). ( b ) Gwl reduces the dose dependence of cycB–Cdk1 for NEBD induction in starfish oocytes. Various amounts of purified cycB–Cdk1, having kinase activities of 2.5–50 fmol P min −1 (each dissolved in a volume of 100 pl; Methods), were injected into immature oocytes along with (magenta squares) or without (green diamonds) active rGwl-WT (6.1 amol in 35 pl solution; see ( a ) above). Kinase defective rGwl-G52S (blue triangles) was used as a control. ( c ) Supplementation of purified cycB–Cdk1 with the endogenous level of Gwl reduced the level of cycB–Cdk1 required for NEBD induction in starfish oocytes by ~75% (from 25.1 to 6.12 fmol P min −1 ). From graphs ( a , b ), the amounts of H1K activity required for 50% NEBD were estimated. ( d ) Supplementation with Gwl transforms cycB–Cdk1 to MPF in Xenopus oocytes. For MPF assay, immature oocytes were injected with purified cycB–Cdk1 at a level of H1K activity, which is insufficient for NEBD induction (60 fmol P min −1 in 0.23 nl), without (green) or with various amounts of active rGwl-WT (magenta, 0.01–1.0 ng in 2.1 nl) or control kinase defective rGwl-G52S (blue, 1.0 ng in 2.1 nl). Neither rGwl-WT nor rGwl-G52S alone (gray, 1.0 or 30 ng in 2.1 nl) induced NEBD. As a positive control, CSF extract (black; H1K activity, 60 fmol P min −1 in 18.4 nl) invariably induced NEBD. ( e ) Gwl is localized mostly in the cytoplasm of immature Xenopus oocytes. Amounts of Gwl were compared by immunoblotting among whole immature oocytes (whole), enucleated immature oocytes (cytoplasm) and isolated GVs (nucleus). Mcm2 and α-tubulin are nuclear and cytoplasmic markers, respectively. Full size image Next, in the frog oocyte system, we performed another type of quantitative analysis to determine whether increasing amounts of Gwl affect the ability of purified cyclin B–Cdk1 to induce the meiotic G2/M-phase transition. The activity level of cyclin B–Cdk1 was first fixed at 60 fmol P min −1 , at an intermediate level where the CSF extract (that is, MPF) induced the G2/M-phase transition invariably, whereas purified cyclin B–Cdk1 alone was completely incapable of promoting NEBD in recipients ( Fig. 1a ). As shown in Fig. 5d , addition of the active rGwl-WT (0.01–1.0 ng) enabled, in a dose-dependent fashion, purified cyclin B–Cdk1 to exhibit M-phase-inducing ability. rGwl alone was unable to promote M-phase even at the maximum 30 ng, an amount of Gwl roughly one order of magnitude lower than that previously reported to induce meiotic G2/M-phase transition when injected into Xenopus oocytes [41] . Thus, Gwl's effect in reducing the level of cyclin B–Cdk1 activity required for the G2/M-phase transition is common to both the frog and starfish oocyte systems. We then examined the localization of Gwl in immature Xenopus oocytes, because enucleation does not severely compromise the appearance of MPF in oocytes of the frog species of Rana pipiens [4] and Xenopus laevis [42] . In immature Xenopus oocytes, most of Gwl was localized in the cytoplasm, although a small fraction was detectable in the nucleus ( Fig. 5e and Supplementary Fig. S5 ). Thus, the contribution of Gwl to MPF through reducing the required amount of cyclin B–Cdk1 is not linked to the nuclear localization of Gwl, but is most likely a general feature of Gwl regardless of its localization. Reduction of cyclin B–Cdk1 is necessary for spindle assembly To address a possible physiological implication of reducing the required level of cyclin B–Cdk1 activity by Gwl, we monitored meiotic spindle assembly and chromosome alignment by imaging microtubules and chromosomes after NEBD in live recipient starfish oocytes. Surprisingly, when purified cyclin B–Cdk1 alone (that is, the excess levels of cyclin B–Cdk1) induced NEBD, the meiotic spindle mostly failed to assemble ( Fig. 6b ; compare with control meiotic spindle formed after 1-MeAde treatment in Fig. 6a ). Some condensed chromosomes congressed to the vicinity of slightly separated centrosomes, although it remains unclear whether all chromosomes did so. As a result, emission of the first polar body was abortive (data not shown). Such failure in spindle assembly was also detectable when Gwl was supplemented to the excess amount of cyclin B–Cdk1 at the injection ( Fig. 6c ). This defect was not a peculiarity of our particular preparation of purified cyclin B–Cdk1, because injection of a large amount of cyclin B mRNA into immature starfish oocytes caused the similar inhibition phenotype (data not shown). In contrast, when either the reduced level of purified cyclin B–Cdk1 along with Gwl ( Fig. 6d ) or control cytoplasmic MPF ( Fig. 6e ) induced NEBD, the meiotic spindle was assembled and chromosomes were aligned on the metaphase plate. 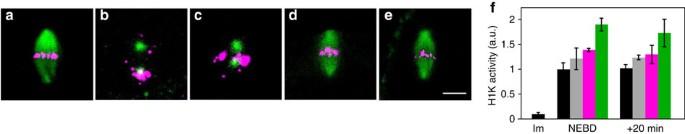Figure 6: Excess cyclin B–Cdk1 is deleterious for spindle assembly in starfish oocytes. (a–e) Meiotic spindle is assembled in starfish oocytes, which have undergone NEBD following injection with the reduced level of cyclin B–Cdk1 plus Gwl, but not in those with the excess level of cyclin B–Cdk1 alone. Live-cell images of microtubules (green) and chromosomes (magenta) for a control 1-MeAde-treated oocyte (a), and oocytes injected with the excess cyclin B–Cdk1 alone (b), the excess cyclin B–Cdk1 plus Gwl (c), the reduced cyclin B–Cdk1 plus Gwl (d) and cytoplasmic MPF (e). Maximum intensity Z projections using ImageJ are shown at a time point equivalent to metaphase of meiosis I. More than ten oocytes from different females were examined for each ofb–e. For injection of purified cyclin B–Cdk1, minimum amounts of kinase activity required for 100% NEBD were estimated to be 50 fmol P min−1for cyclin B–Cdk1 alone (excess) and 15 fmol P min−1for cyclin B–Cdk1 (reduced) plus Gwl, respectively (each dissolved in a volume of 100 pl for cyclin B–Cdk1). The same amount of active rGwl-WT (10 amol in 50 pl) was injected inc,d. All figures were taken at the same magnification, and bar indicates 10 μm. (f) Comparison of Cdk1 activity contained in oocytes after NEBD. Levels of H1K activity contained in starfish oocytes were measured at NEBD and NEBD plus 20 min (equivalent to metaphase of meiosis I) after injection with the excess cyclin B–Cdk1 alone (green), the reduced cyclin B–Cdk1 plus Gwl (magenta) or cytoplasmic MPF (gray), or after control treatment with 1-MeAde (black). Im indicates immature oocytes. Each H1K activity was measured from an oocyte. Bars indicate s.e. of six separate experiments. Figure 6: Excess cyclin B–Cdk1 is deleterious for spindle assembly in starfish oocytes. ( a – e ) Meiotic spindle is assembled in starfish oocytes, which have undergone NEBD following injection with the reduced level of cyclin B–Cdk1 plus Gwl, but not in those with the excess level of cyclin B–Cdk1 alone. Live-cell images of microtubules (green) and chromosomes (magenta) for a control 1-MeAde-treated oocyte ( a ), and oocytes injected with the excess cyclin B–Cdk1 alone ( b ), the excess cyclin B–Cdk1 plus Gwl ( c ), the reduced cyclin B–Cdk1 plus Gwl ( d ) and cytoplasmic MPF ( e ). Maximum intensity Z projections using ImageJ are shown at a time point equivalent to metaphase of meiosis I. More than ten oocytes from different females were examined for each of b – e . For injection of purified cyclin B–Cdk1, minimum amounts of kinase activity required for 100% NEBD were estimated to be 50 fmol P min −1 for cyclin B–Cdk1 alone (excess) and 15 fmol P min −1 for cyclin B–Cdk1 (reduced) plus Gwl, respectively (each dissolved in a volume of 100 pl for cyclin B–Cdk1). The same amount of active rGwl-WT (10 amol in 50 pl) was injected in c , d . All figures were taken at the same magnification, and bar indicates 10 μm. ( f ) Comparison of Cdk1 activity contained in oocytes after NEBD. Levels of H1K activity contained in starfish oocytes were measured at NEBD and NEBD plus 20 min (equivalent to metaphase of meiosis I) after injection with the excess cyclin B–Cdk1 alone (green), the reduced cyclin B–Cdk1 plus Gwl (magenta) or cytoplasmic MPF (gray), or after control treatment with 1-MeAde (black). Im indicates immature oocytes. Each H1K activity was measured from an oocyte. Bars indicate s.e. of six separate experiments. Full size image Quantitative comparison indicates that the level of Cdk1 activity contained in starfish oocytes at NEBD was at most twofold higher when injected with the excess level of cyclin B–Cdk1 alone, and 1.5-fold higher when injected with the reduced level of cyclin B–Cdk1 plus Gwl, than when treated with 1-MeAde or injected with cytoplasmic MPF ( Fig. 6f ; see also Fig. 6A in ref. 27 ). In oocytes injected with the excess cyclin B–Cdk1 alone, Cdk1 activity remained at the elevated levels at least for 20 min when the control oocytes reached metaphase of meiosis I ( Fig. 6f ), but thereafter, Cdk1 became finally inactivated (data not shown). Although the twofold higher levels of activity do not appear to be extraordinary, the observed defects may be caused on the background that the endogenous levels of cyclin B–Cdk1 activity in meiosis I are much higher than those in meiosis II and in M-phase of cleavage cycles (for example, ref. 35 ). Thus, the excess amount of cyclin B–Cdk1 is deleterious for spindle assembly even though it can induce NEBD. Gwl contributes to formation of the spindle with properly aligned chromosomes after NEBD through reducing the amount of cyclin B–Cdk1 required for NEBD. MPF was originally defined as a transferable activity that can induce M-phase in recipient cells, implying that MPF's presence in donor cells can be verified only when its activity is detectable in recipient cells. Today, MPF is assumed to describe an activity that exhibits its effect in donor cells; furthermore, MPF is consistently equated with cyclin B–Cdk1. We show here that a major gap exists between the original functional definition of MPF and the relatively imprecise ways in which this term is currently used. We have found that in two different species (a vertebrate and an invertebrate), Gwl is a novel component of the maturation-promoting factor activity that can be transferred from donor to recipient oocytes. MPF defined by the classical functional assay clearly consists of at least two separate components: the kinases cyclin B–Cdk1 and Gwl. The general view that MPF is identical to cyclin B–Cdk1 must therefore be altered. We believe it is most fruitful to consider MPF as a complete system that couples activation of the cyclin B–Cdk1 kinase, which executes entry into M-phase with concomitant suppression of the phosphatase (PP2A-B55) that counteracts the cyclin B–Cdk1 driver. The linkage of these events, mediated through Gwl, allows cyclin B–Cdk1 to trigger all aspects of M-phase (NEBD and spindle assembly) in recipient cells at reduced, physiological levels. Our results identify Gwl as an essential component of MPF in one specialized type of germline cell (that is, the oocyte), but Gwl may be a critical constituent of MPF in the somatic cells of higher eukaryotes as well. To our knowledge, the literature provides no evidence that the simple introduction of active cyclin B–Cdk1 leads to entry into M-phase in somatic cells [43] , [44] . Considering that Gwl is also nuclear and its depletion results in G2-phase arrest in both Drosophila [20] and human somatic cells [45] , Gwl could be an essential component of MPF in somatic cells as well. How then does Gwl reduce the required amount of cyclin B–Cdk1 activity? We confirmed that Gwl phosphorylates starfish Ensa/Arpp19 to inhibit PP2A-B55 in vitro (data not shown), as already shown in other systems [22] , [23] . Gwl and its target(s) Ensa/Arpp19 influence the G2/M-phase transition not only by opposing the dephosphorylation of downstream cyclin B–Cdk1 target proteins, but also by participating in the well-known autoregulatory loop for cyclin B–Cdk1 itself [21] , [41] , [46] ( Fig. 7 ). In this loop, cyclin B–Cdk1 promotes its own activation through positive feedback to Cdc25 and negative feedback to Myt1 and Wee1. Many of the phosphorylation events responsible for both positive and negative feedback in the loop are directly catalysed by cyclin B–Cdk1, but are in large part opposed by PP2A-B55. Cyclin B–Cdk1 activates Gwl [21] , which in turn suppresses PP2A-B55 through Ensa/Arpp19, whereas activation of Gwl by cyclin B–Cdk1 might be opposed by PP2A-B55. In this way, cyclin B–Cdk1-driven phosphorylations of Cdc25, Myt1 and Wee1 can be maintained during M-phase entry. The cyclin B–Cdk1–Gwl pathway (that is, MPF) therefore constitutes a core of the autoregulatory loop in donor cells ( Fig. 7 ). This core element is key to autocatalysis of the loop as a whole in recipient cells as well, because transfer of MPF yields all relevant M-phase-specific changes. In particular, after transfer of MPF, the introduced cyclin B–Cdk1 is opposed by PP2A-B55 in making and maintaining Gwl active in recipient cells. In that case, the co-injected active Gwl might suppress PP2A-B55 and make it easier for cyclin B–Cdk1 to activate Gwl in recipient cells. In addition, the introduced cyclin B–Cdk1 is directly attacked by Myt1, which is highly active in recipient immature oocytes [27] , [29] . The co-injection of activated Gwl could help, through the autoregulatory loop, the introduced cyclin B–Cdk1 to escape at least partially from the inactivation in recipient cells. Together, the co-injection of activated Gwl could enhance autocatalysis of the loop and hence reduces the amount of cyclin B–Cdk1 activity required for injection. This also explains the reason why cytoplasm from enucleated starfish oocytes, which contain endogenous, that is, unexcess levels of cyclin B–Cdk1 but not Gwl, exhibits no MPF activity. 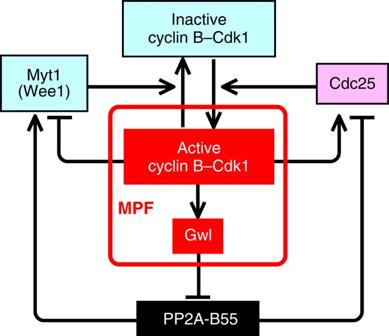Figure 7: MPF as a core component in the autoregulatory loop for cyclin B–Cdk1 activation. Cyclin B–Cdk1 is by itself very inefficient in triggering the autoregulatory loop in recipient oocytes, but MPF, consisting of both cyclin B–Cdk1 and Gwl, can efficiently initiate the activation loop, leading to full activation of cyclin B–Cdk1 in recipients. Figure 7: MPF as a core component in the autoregulatory loop for cyclin B–Cdk1 activation. Cyclin B–Cdk1 is by itself very inefficient in triggering the autoregulatory loop in recipient oocytes, but MPF, consisting of both cyclin B–Cdk1 and Gwl, can efficiently initiate the activation loop, leading to full activation of cyclin B–Cdk1 in recipients. Full size image Our results also reveal the physiological relevance for reducing the required level of cyclin B–Cdk1 by Gwl. The excess level of Cdk1 activity has deleterious effect on spindle assembly after NEBD, even though it can induce NEBD. Although Gwl is known to enhance proper alignment of chromosomes on the spindle in the absence of exogenous cyclin B–Cdk1 (refs 20 , 45 ), our study points out another aspect that Gwl contributes to proper assembly of the meiotic spindle through reducing the levels of cyclin B–Cdk1 activity required for NEBD. Gwl thus coordinates NEBD and spindle assembly at entry into M-phase. Although chromosome misalignment is detectable in human cultured cells in which nondegradable cyclin B1 is expressed at levels equivalent to the endogenous levels [47] , and different levels of cyclin B–Cdk1 activity trigger and regulate different mitotic events to coordinate mitosis [48] , [49] , the present observation might be, so far we know, the first to show relationship between the levels of Cdk1 activity and spindle assembly. In the presence of the excess Cdk1 activity, microtubules do not appear to be properly regulated to assemble the spindle, even though they can possibly capture some chromosomes. It is plausible that the excess cyclin B–Cdk1 activity leads to aberrant phosphorylation of regulators of spindle assembly, thereby altering their function. Curiously, Gwl is not essential for the meiotic G2/M transition and full activation of cyclin B–Cdk1 in starfish oocytes treated with 1-MeAde ( Figs 1c,d and 3d,e ), even though Gwl is absolutely required for detectable MPF when cytoplasm from these oocytes is used as a donor ( Figs 3f and 4b,c ). These observations contrast with previous report that cyclin B–Cdk1 fails to become active in Gwl-depleted cycling extracts from Xenopus eggs [21] . The inconsistency, at least in part, probably reflects the fact that the starfish experiments examine entry into meiosis-I, whereas the frog cycling extracts mimic mitotic divisions in some aspects. In meiosis I, extracellular maturation-inducing hormone triggers the G2/M-phase transition absolutely upstream of the regulatory components for cyclin B–Cdk1 activation [27] . Indeed, 1-MeAde causes inhibition of Myt1 activity via activation of Akt/PKB before, and in the absence of, cyclin B–Cdk1 activation [29] . Our preliminary observations suggest that Myt1 phosphorylation by Akt/PKB is insensitive to PP2A-B55. 1-MeAde may in this way tip the balance of activities between cyclin B–Cdk1 and PP2A-B55 toward full activation of cyclin B–Cdk1 in enucleated meiosis I oocytes of starfish devoid of Gwl. In contrast, MPF, which is injected into immature oocytes, is considered as a midway initiator on the autoregulatory loop for cyclin B–Cdk1 activation ( Fig. 7 ) in the absence of absolutely upstream stimulus (for example, maturation-inducing hormone). This difference may explain the different dependence on Gwl between 1-MeAde- and MPF-induced meiotic G2/M-phase transition. Another fascinating possibility is that cells may have a secondary autoregulatory loop for cyclin B–Cdk1 activation that is independent of Gwl, although the key element of this putative loop should not be transferable into recipient oocytes for detection of MPF activity. We are thus attempting to determine whether PP2A-B55 is suppressed after 1-MeAde addition in enucleated starfish oocytes. Starfish oocytes and cyclin B–Cdk1 purification Immature oocytes of the starfish, Asterina pectinifera (renamed Patiria pectinifera in the 2007 NCBI Taxonomy Browser), were prepared as described [35] , and treated with 1 μM 1-MeAde [25] to induce meiotic maturation at 20 °C in artificial sea water. Microinjection, enucleation and cytoplasmic transfer for MPF assay were performed as described [5] , [28] . The volume of an oocyte was calculated to be 3.0 nl by measuring the diameter under a microscope. For assay of cytoplasmic MPF, 250 pl of cytoplasm was transferred from maturing oocytes 25–50 min after 1-MeAde addition to untreated immature oocytes, and GVBD in recipient oocytes was inspected at 60 min after the injection. The volume of cytoplasmic MPF that induces NEBD in 50% of recipient oocytes was found to be 105 pl ( Fig. 5a ). When recombinant Gwl was injected along with enucleated oocyte cytoplasm ( Fig. 4c ) or along with purified cyclin B–Cdk1 ( Fig. 5b ) into immature oocytes, each of these was separated by silicon oil in a single glass micropipette. Active cyclin B–Cdk1 was purified from meta-I starfish oocytes by Suc1-beads as described [27] . The use of all animals (starfish, frogs and rabbits) complied with our institute regulations. Xenopus oocytes and their extracts Female frogs ( Xenopus laevis ) were primed with injection of 100 U of P-Mex (Yell Pharmaceutical) 4 days before the preparation of defolliculated oocytes by previously described methods [50] . Oocytes were washed several times with Modified Barth's saline (88 mM NaCl, 1 mM KCl, 2.4 mM NaHCO 3 , 0.82 mM MgSO 4 , 0.32 mM Ca(NO 3 ) 2 , 0.41 mM CaCl 2 , 10 mM HEPES, pH 7.5). Stage VI oocytes were injected using Nanoject II (Drummond Scientific) with CSF extracts, purified starfish cyclin B–Cdk1 and recombinant starfish Gwl, or treated with 5 μg ml −1 of progesterone to induce maturation. Injected or progesterone-treated oocytes were cultured in Modified Bath's saline (MBS) at 23 °C, and GVBD was recognized 3 h later as a white spot appearing at the animal pole and then verified by dissection of the oocytes after boiling [51] . To prepare CSF extracts [26] , the primed frogs were injected with 100 U of Gonatropin (Aska Pharmaceutical), and 12 h later, ovulated eggs were collected and dejellied [51] . One hundred unfertilized meta-II eggs were recovered in 250 μl of β-glycerophosphate extraction buffer (BG-EB) (80 mM β-glycerophosphate, 20 mM EGTA, 5 mM MgCl 2 , 20 mM HEPES-KOH, pH 7.3) and homogenized by pipetting up and down with a yellow tip. After centrifugation (12,000 g for 1 min, 2 °C), the cytoplasmic fraction was collected, divided into aliquots, frozen in liquid nitrogen and stored at −80 °C. Although CSF extracts contain Wee1A, this might have no impact on MPF activity, because Wee1A is inactive in CSF extracts and undetectable in recipient immature frog oocytes [52] . Cytoplasmic and GV fractions were obtained after manual enucleation in 70% Marc's modified Ringer's (MMR) (100% MMR: 100 mM NaCl, 2 mM KCl, 1 mM MgCl 2 , 2 mM CaCl 2 , 0.1 mM EDTA, 5 mM HEPES, pH 7.8). Ten intact or enucleated oocytes were recovered in 100 μl of BG-EB. Oocyte extracts were prepared as above, supplemented with 1/4 volume of 4× Laemmli's sample buffer (LSB) and boiled for 5 min. Ten GV were recovered in 20 μl of 70% MMR; an equal volume of 2×LSB was added and the mixture boiled. Quantitative measurement of H1K activity To measure H1K activity quantitatively in meta-I starfish oocytes, ten oocytes (40 min after 1-MeAde addition) were washed with an extraction buffer (80 mM β-glycerophosphate, 20 mM EGTA, 100 mM KCl, 15 mM MgCl 2 , 100 mM sucrose, 1 mM dithiothreitol, protease inhibitor cocktail (Complete EDTA-free, Roche), pH 7.3), recovered in 1 μl of the extraction buffer and frozen in liquid nitrogen. The thawed preparation was mixed with 9 μl of H1 reaction solution (final concentration in 10 μl of the mixture: 0.3 mg ml −1 histone H1, 100 μM ATP, 2 mM MgCl 2 , 10 mM Tris–HCl, pH7.5, 5.6 MBq ml −1 [γ- 32 P]ATP) and incubated for 30 min at 25 °C. The reaction was terminated by addition of 5 μl 3×LSB containing 5 mM EDTA and boiling for 5 min. Seven microlitre of the sample was fractionated by SDS–polyacrylamide gel electrophoresis (12.5%), and phosphorylation of histone H1 was quantified with liquid scintillation counting. The CSF extracts and purified cyclin B–Cdk1 were diluted appropriately with BG-EB or Cdk1 buffer (80 mM β-glycerophosphate, 20 mM EGTA, 15 mM MgCl 2 , 1 mM dithiothreitol, 10% sucrose, 0.1% NP-40, 0.1% bovine serum albumin, pH 7.3), respectively. H1K activity in 1 μl each of CSF extracts and of purified cyclin B–Cdk1 was measured as described above. H1K activity was finally calculated as an activity that catalyses the transfer of phosphate from ATP to histone H1 per minute per volume. At least three independent measurements were performed using different batches of frogs and starfish to obtain the data shown in Figs 1a,b and 5a–d . Typically, to compare the meiotic G2/M-phase transition-inducing activity, 18.4, 13.8, 9.2, 4.6 and 2.3 nl each of CSF extracts (frog MPF; H1K activity, 1.57 pmol P min −1 μl −1 ) or cyclin B–Cdk1 (H1K activity, 21.7 pmol P min −1 μl −1 ) were injected into immature Xenopus oocytes ( Fig. 1a ); and 200, 150, 100 and 50 pl each of the cytoplasm of meta-I starfish oocytes (starfish MPF; H1K activity, 35 pmol P min −1 μl −1 ) or cyclin B–Cdk1 (H1K activity, 230 pmol P min −1 μl −1 ) were injected into immature starfish oocytes ( Fig. 1b ). To examine the effect of Gwl on the meiotic G2/M-phase transition-inducing activity of purified cyclin B–Cdk1 in starfish oocytes, the purified cyclin B–Cdk1 preparation (H1K activity, 517 pmol P min −1 μl −1 ) was variously diluted to a final volume of 100 pl, each containing 2.5–50 fmol P min −1 of H1K activity ( Fig. 5b,c ). In this experiment, cytoplasm of meta-I starfish oocytes (starfish MPF) contained 24 pmol P min −1 μl −1 of H1K activity, and accordingly, 105 pl of cytoplasm (that is, the amount that induces 50% NEBD in recipients) was calculated to contain 2.5 fmol P min −1 of H1K activity ( Fig. 5a,c ). To examine the effect of Gwl in Xenopus oocytes, the amount of H1K activity was fixed at 60 fmol P min −1 in both CSF extracts (in 18.4 nl) and purified cyclin B–Cdk1 (in 2.3 nl; Fig. 5d ). IgG introduction into GV To test the ability for ZZ-IBB to introduce IgG into GVs, ZZ-IBB was incubated with Alexa 488-conjugated Donkey anti-rabbit IgG (Invitrogen) for 30 min on ice, and then injected into cytoplasm of immature starfish oocytes. Accumulation of Alexa 488-IgG into the GVs of the oocytes was observed with a confocal microscope (Olympus). To inhibit Gwl activity in vivo , 600 pg anti-Gwl-C antibody and 800 pg ZZ-IBB were incubated together for 30 min on ice, and then injected into the cytoplasm of immature oocytes. Live-cell images of microtubules and chromosomes To monitor meiotic spindle assembly and chromosome alignment, each immature starfish oocyte was injected with both 2% oocyte volume of HiLyte-488-labelled porcine brain tubulin (~2 mg ml −1 ; Cytoskeleton Inc., TL488M-A) in G-buffer (100 mM PIPES-KOH, pH 6.9, 1 mM MgSO 4 , 1 mM EGTA, 1 mM GTP) and with 1% oocyte volume of Alexa-568-labelled histone H1 in PBS (prepared at ~1 mg ml −1 using Histone H1 protein (Roche) and Alexa-568 protein labelling kit (Molecular Probes)). Live oocytes were observed with an Olympus Fluoview FV1000 confocal microscope using a water-immersion objective lens (X40). Several sliced images (obtained during 20–30 min after NEBD, which corresponds to metaphase of meiosis I) were projected into a single image by maximum intensity Z projections of ImageJ ( http://rsb.info.nih.gov/ij/ ). How to cite this article: Hara, M. et al . Greatwall kinase and cyclin B-Cdk1 are both critical constituents of M-phase promoting factor. Nat. Commun. 3:1059 doi: 10.1038/ncomms2062 (2012).